Scanning-aperture trapping and manipulation of single charged nanoparticles Although trapping and manipulation of small objects have been of interest for a range of applications and many clever techniques have been devised, new methods are still in great demand for handling different materials and geometries. Here, we report on an electrostatic trap that is created in an aqueous medium between the aperture of a nanopipette and a glass substrate without the need for external potentials. After a thorough characterization of the trapping conditions, we show that we can displace or release a particle at will. Furthermore, we demonstrate trapping and manipulation of nanoparticles and lipid vesicles attached to lipid bilayers, paving the way for controlled studies of forces and diffusion associated with biological membranes. We expect the technique to find interesting applications also in other areas such as optonanofluidics and plasmonics. Over the past three decades, scientists have continually developed and improved methods for trapping small objects, especially for applications in biosciences [1] , [2] , [3] , [4] , [5] , [6] . Nevertheless, many important challenges remain and no single method has been able to satisfy all requirements. One central goal is the contact-free trapping of ever smaller particles down to single proteins or clusters for times beyond seconds. The most celebrated trapping technique, the optical tweezer [2] , [3] , loses its effectiveness in this effort because the dipole force scales as the third power of the particle size so that trapping a particle of 10 nm diameter requires about a million times more intensity than the commonly trapped micron-sized particles, leading to concerns of photodamage [7] . A new trapping method uses field-free electrostatic polarization of glass surfaces in an aqueous environment [8] . By tailoring the local geometry at the nanometre scale, one creates an attractive three-dimensional potential for negatively-charged nanoparticles, while the depth of the trap can be adjusted by varying the geometry, number of charges and ion concentration in the buffer. This method has been used for long-time (minutes to hours) and orientation-dependent trapping of metallic nanoparticles, polymer beads and lipid vesicles with diameters down to 20 nm (refs 8 , 9 ). A crucial advantage of the technique is that the potential depth depends only on the electric charge and not on the mass or size of the object. Another key benefit is that one does not require any external influences such as applied fields or feedback signals although the method can be easily combined with other techniques. The existing reports have used a lab-on-chip approach [8] , [9] , [10] , in which fixed nanoscopic indentations are fabricated on a substrate using electron beam lithography. In this work, we extend this powerful technique to open-access geometries in an experimental arrangement that is commonly available in laboratories. By using scannable nanopipettes, which have long been employed for diverse biophysical [11] , [12] and nanotechnological [13] , [14] , [15] investigations, we demonstrate versatile manipulation of nanoparticles with promising applications in the study of biological membranes. Although in this work we restrict ourselves to negative surface charges and therefore traps for negatively charged particles, the method can be generalized if one treats the glass surfaces involved with appropriate materials such as aminosilanes [16] . 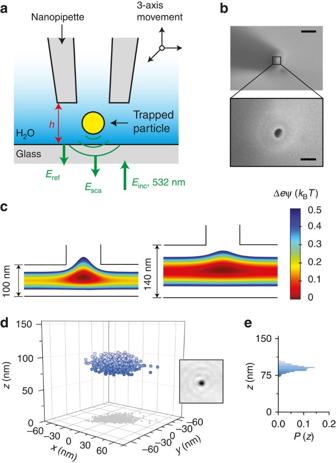Figure 1: Scanning-aperture electrostatic trap. (a) Schematics of a particle trapped between a scannable nanopipette and a substrate in an aqueous bath. The quantitiesEinc,ErefandEsca(green arrows) signify the electric fields associated with the incident, reflected and scattered beams, respectively. The optical elements involved in the iSCAT detection are not shown. (b) Field emission scanning electron microscope image (scale bar, 5 μm) and its zoom of a glass nanopipette end (scale bar, 200 nm). (c) The calculated electrostatic potential of a point charge in two different pipette-substrate gaps of 100 and 140 nm. (d) Three-dimensional representation of 1,000 positions of a GNP recorded at a rate of 1.9 kHz. The inset shows an example of an iSCAT image recorded in one frame. (e) The histogram of the particle axial positions. Experimental considerations Figure 1a depicts the core of our experimental arrangement. A heat-pulled glass nanopipette is held in a three-dimensional stage with nanometre (piezo scanner) and micrometre (translation stage) displacement capabilities. Figure 1b displays an electron microscope image of a nanopipette with an aperture diameter of about 100 nm. We estimate the number density of surface charges on the substrate and the pipette to be σ s ≈10 16 e m −2 , arising from spontaneous ionization in water [17] . In Fig. 1c , we show the calculated electrostatic potential of a point charge for two different pipette-substrate gaps ( h ) obtained by solving the nonlinear Poisson–Boltzmann equation numerically (COMSOL Multiphysics 4.2a). These confirm that potentials as deep as several k B T can be obtained for only a few elementary charges e within a geometrical indentation of tens of nanometres. More insight into the axial profile of the potential can be found in Supplementary Fig. 1 . Figure 1: Scanning-aperture electrostatic trap. ( a ) Schematics of a particle trapped between a scannable nanopipette and a substrate in an aqueous bath. The quantities E inc , E ref and E sca (green arrows) signify the electric fields associated with the incident, reflected and scattered beams, respectively. The optical elements involved in the iSCAT detection are not shown. ( b ) Field emission scanning electron microscope image (scale bar, 5 μm) and its zoom of a glass nanopipette end (scale bar, 200 nm). ( c ) The calculated electrostatic potential of a point charge in two different pipette-substrate gaps of 100 and 140 nm. ( d ) Three-dimensional representation of 1,000 positions of a GNP recorded at a rate of 1.9 kHz. The inset shows an example of an iSCAT image recorded in one frame. ( e ) The histogram of the particle axial positions. Full size image To visualize the trajectory of a trapped particle, we employ a home-built inverted optical microscope under the stage of our piezo scanning nanopipette. We image the particle motion on a camera by monitoring the interference between the laser beam reflected from the substrate and the light scattered by the nanoparticle (see Fig. 1a ). An example of the images obtained by this interferometric scattering (iSCAT) detection method [18] is displayed in the inset of Fig. 1d . By fitting the central image spot with a Gaussian profile, we localize the particle in the lateral plane. Furthermore, the interferometric variation of the contrast in the axial direction gives access to the axial displacement of the particle with nanometre accuracy [19] . Technical details of iSCAT imaging are found in the Methods section and ref. 19 . Figure 1d provides a three-dimensional map of the locations of a gold nanoparticle (GNP) with a diameter of 60 nm and negative charge of ~−93 e in a trap created by a pipette aperture of 100 nm and a gap h ~150 nm. To measure the latter, the pipette was first brought into contact with the glass substrate, where the iSCAT signal of the pipette end does not change anymore, and then retracted using the reading of the piezoelectric stage. Figure 1d,e reveal the strong lateral (40 nm) and axial (15 nm) confinements of the particle. Calibrated measurements confirm that the particle levitates at about a height of 90 nm above the substrate, that is, without contact with any surfaces. If we approximate the trap potential with a harmonic profile, we can deduce a radial trap stiffness ( k r ) from the distribution of the particle positions. For the example presented in Fig. 1 , one arrives at k r ~15 μN m −1 equivalent to 15 fN nm −1 . We note in passing that the lateral asymmetry of the trap (see projection in Fig. 1d ) is caused by the elongated shape of the pipette aperture (see Fig. 1b ). Quantitative analysis of trap performance To obtain a quantitative understanding of the trap characteristics as a function of h , we need to take into account the finite size of the particle (as opposed to the simpler point-charge treatment in Fig. 1c ). Here, we calculated the Helmholtz free energy F of the system including the GNP by summing the electrostatic field energies and entropies over all charges in three dimensions [20] . 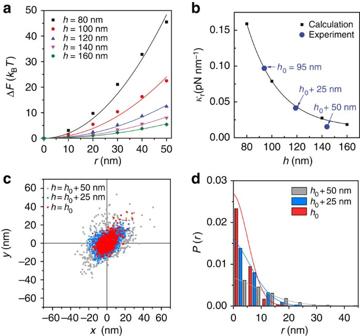Figure 2: The effect of nanopipette height. (a,b) Dependence of trapping free energy on a tunable gaph. (a) Radial free energy profiles calculated along the contour of the axial energy minimum with different gapsh. (b) Calculated (black) and measured (blue) values of radial trapping stiffness,krfor differenth. (c) Transverse (x-y) positions of a single 60 nm GNP trapped by a nanopipette at different gapsh0~100 nm (red),h0+25 nm (light blue), andh0+50 nm (grey) in 0.04 mM electrolyte. Ath0+75 nm, the particle escaped from the trap. Each scatter plot was obtained from iSCAT images of 1,000 frames at a rate of 1.9 kHz. (d) Radial probability histograms of the trapped particle in each case. Figure 2a illustrates the radial free energy profiles for a 60 nm GNP (~−93 e ) and different gaps of 80–160 nm. A simple estimate of the trapping stiffness k r according to F ( r )= k r r 2 /2 is represented by the square symbols and black line in Fig. 2b following an exponential behaviour of k r ~exp(−0.04 h ). Figure 2: The effect of nanopipette height. ( a , b ) Dependence of trapping free energy on a tunable gap h . ( a ) Radial free energy profiles calculated along the contour of the axial energy minimum with different gaps h . ( b ) Calculated (black) and measured (blue) values of radial trapping stiffness, k r for different h . ( c ) Transverse (x-y) positions of a single 60 nm GNP trapped by a nanopipette at different gaps h 0 ~100 nm (red), h 0 +25 nm (light blue), and h 0 +50 nm (grey) in 0.04 mM electrolyte. At h 0 +75 nm, the particle escaped from the trap. Each scatter plot was obtained from iSCAT images of 1,000 frames at a rate of 1.9 kHz. ( d ) Radial probability histograms of the trapped particle in each case. Full size image Aside from its ease of fabrication, a remarkable advantage of our experimental strategy over a chip-based approach is the possibility of an in situ and dynamic control of the trap stiffness by instant variation of the nanopipette height. To demonstrate this effect, in Fig. 2c,d (see also Supplementary Movie 1 ) we present the trap performance for different values of h = h 0 (red), h 0 +25 nm (light blue) and h 0 +50 nm (grey), whereby h 0 was measured to be about 100 nm. It is clear from the behaviour of the lateral position map of the particle and the probability density distribution [8] P ( r ) that increasing h renders the trap shallower. In fact, the particle quickly escaped from the gap when h was increased to h 0 +75 nm. The good agreement of the experimental values of k r (see round symbols in Fig. 2b ) and the theoretical prediction lets us deduce h 0 ~95 nm, which confirms our independent measurement of h 0 ~100 nm mentioned above. Another important trap parameter is the ion concentration ( C ) because the electrostatic potential near a charged surface in a solution decays exponentially with a Debye length, which is proportional to . To this end, a higher ion strength screens surface charges and makes trapping weaker. 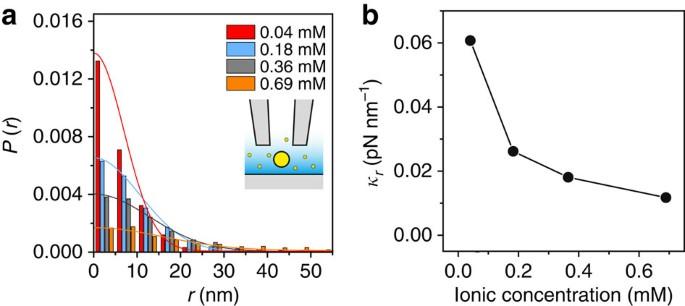Figure 3: Effect of ion strength. (a) Radial probability histograms of a GNP (60 nm) by a nanopipette ath~120 nm for different ion strengths. (b) Dependence of trap stiffness on ion concentration. Figure 3 illustrates the radial probability density distributions of the same single GNP as above for different ionic strengths of 0.04, 0.18, 0.36 to 0.69 mM obtained by incremental in situ addition of NaCl to the system at h ~120 nm. This clearly shows that the distribution of the particle motion becomes broader as the ionic strength increases. The trap stiffness decreases from 60 to 10 fN nm −1 as the ionic strength increases from 0.04 to 0.69 mM. In addition to validating the electrostatic nature of the potential, these measurements indicate that our trapping scheme could be used to detect changes in the local ion strength. We remark that the weaker trap stiffness at higher ion concentrations, which poses a challenge for operation in physiological buffer, can be compensated in smaller traps. Indeed, calculations show the feasibility of single protein trapping if the gap is reduced to the order of 10 nm. Although on-chip nanofabrication of gaps at this scale is a nontrivial task, scanning probe technology provides a straightforward way to achieve such small pipette-substrate separations. Figure 3: Effect of ion strength. ( a ) Radial probability histograms of a GNP (60 nm) by a nanopipette at h ~120 nm for different ion strengths. ( b ) Dependence of trap stiffness on ion concentration. 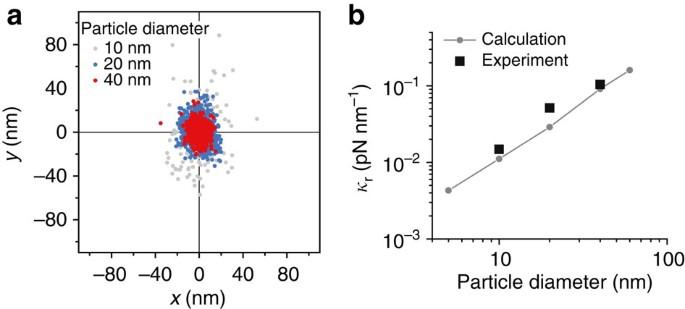Figure 4: Trapping smaller particles. (a) Transverse position of single 40, 20 and 10 nm GNPs confined by a nanopipette ath~75 nm. (b) Measured and calculated trap stiffness for the particles studied ina. Full size image Figure 4 shows the ability of our method in creating tight trap geometries and thus confining particles as small as 10 nm. In Fig. 4a , we display the position maps of particles with diameters of 40, 20 and 10 nm (~−67 e , −27 e and −11 e , respectively) at h ~75 nm. It is clear that smaller GNPs with fewer charges experience shallower traps in the same nanogeometry. Figure 4b presents a very good agreement between the measured and computed values of the radial trap stiffness as a function of particle size (also see radial free energy profiles in Supplementary Fig. 2 ). It is interesting to note that the charges on many proteins are considerably larger than that of a 10 nm GNP used in our demonstration (see Supplementary Table 1 ). Figure 4: Trapping smaller particles. ( a ) Transverse position of single 40, 20 and 10 nm GNPs confined by a nanopipette at h ~75 nm. ( b ) Measured and calculated trap stiffness for the particles studied in a . Full size image Trapping and manipulation of nanoparticles bound to lipid membranes The scanning probe feature of our trapping scheme makes it possible to manipulate particles bound to interfaces. As a particularly interesting case, we have examined the applicability of our trap to investigations of phospholipid membranes (see Fig. 5 ). Here, we prepared 1 mol% ganglioside GM1 in a 1,2-dioleoyl-sn-glycero-3-phosphocholine (DOPC) bilayer on a cover glass. GNPs (diameter 40 nm) coated with cholera toxin B were then added, which could bind to the GM1 lipids in the bilayer [18] and undergo lateral random motion governed by the diffusion of the GM1 lipids in the membrane. We employed iSCAT to track the GNPs. Once a given particle was targeted, we used the piezoelectric scanner of the nanopipette to chase and trap it as illustrated by the sequence of Fig. 5b–d (see also Supplementary Movie 2 ). In addition, the trapped particle can be steered laterally to a new location (see Supplementary Movie 3 ). The iSCAT images in Fig. 5e show the start and end positions of a particle pulled over 1.6 μm and then released by lifting the nanopipette, while the graph displays its full trajectory. We point out that Jönsson et al. [21] have recently also presented a nanopipette-based trap that operates by attracting molecules attached to membranes under a negative pressure. This interesting approach is complementary to our method in that it is nonspecific in its selection of the molecules to be trapped. 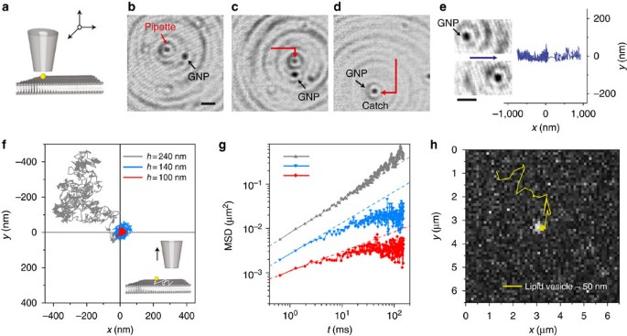Figure 5: Applications to lipid systems. (a–g) Direct manipulation of a single GNP on a phospholipid membrane consisting of 1 mol% GM1 in DOPC. (a) The experimental arrangement. (b–d) A series of iSCAT images for catching a GNP. (scale bar, 1 μm.) (b) Images of the pipette end and a nearby particle. (c) The nanopipette is brought closer to the particle, which has moved since (b). (d) The nanopipette has caught up with the particle. (e) Two iSCAT images before and after lateral displacement of 1.6 μm. The blue trace displays the trajectory of the GNP during the displacement. (scale bar, 1 μm.) (f) Lateral trajectories of a trapped GNP at different nanopipette heights. (g) The mean square displacements with time corresponding to the trajectories in (f). The trapped particle (red and blue traces) undergoes subdiffusive motion. (h) Lateral trajectory of a lipid vesicle (diameter ~50 nm) bound to the membrane, leading to trapping under the nanopipette. In this experiment, the vesicle was labelled with fluorescent dyes (Atto532). Figure 5: Applications to lipid systems. ( a – g ) Direct manipulation of a single GNP on a phospholipid membrane consisting of 1 mol% GM1 in DOPC. ( a ) The experimental arrangement. ( b – d ) A series of iSCAT images for catching a GNP. (scale bar, 1 μm.) ( b ) Images of the pipette end and a nearby particle. ( c ) The nanopipette is brought closer to the particle, which has moved since ( b ). ( d ) The nanopipette has caught up with the particle. ( e ) Two iSCAT images before and after lateral displacement of 1.6 μm. The blue trace displays the trajectory of the GNP during the displacement. (scale bar, 1 μm.) ( f ) Lateral trajectories of a trapped GNP at different nanopipette heights. ( g ) The mean square displacements with time corresponding to the trajectories in ( f ). The trapped particle (red and blue traces) undergoes subdiffusive motion. ( h ) Lateral trajectory of a lipid vesicle (diameter ~50 nm) bound to the membrane, leading to trapping under the nanopipette. In this experiment, the vesicle was labelled with fluorescent dyes (Atto532). Full size image A topic of great interest in membrane biophysics is the quantitative understanding of diffusion of lipids and proteins in confined geometries [22] . In addition to the limited spatial resolution of the existing optical methods, fast movements corresponding to diffusion constants of the order of μm 2 s −1 make it a major challenge to interrogate the nanoscopic details of binding and unbinding events of bioparticles such as viruses [18] , [23] . Confining a particle over a few tens of nanometres would allow long-time study of the interaction between the particle surface and the membrane. In order to demonstrate the applicability of our technique to these problems, in Fig. 5f we display the trajectories of a cholera toxin B covered GNP trapped in gaps of 100 nm (red) and 140 nm (blue). Plotting the mean square displacement as a function of time ( t ) on a logarithmic scale reveals a clear deviation from a line (see Fig. 5g ), thus, revealing a subdiffusive motion [24] . As expected, the grey traces in Fig. 5f,g show that the particle undergoes normal diffusion upon escape from the trap when the gap was increased to 240 nm. Another system of interest in modern biophysics is fusion and budding of lipid vesicles with and out of lipid membranes [25] . In Fig. 5h , we present the trapping trajectory of a small negatively charged unilamellar vesicle (diameter about 50 nm) anchored to a supported lipid bilayer via biotin–avidin chemistry [26] (see Methods). Combination of the strong lateral confinement within 20 nm ( Supplementary Movie 4 ) with the ability to control the height of the trapped particle opens the door for quantitative and controlled studies of vesicle–membrane interactions [27] . The advantages of field-free and non-contact geometry-induced electrostatic trapping have been discussed in previous works [8] , [10] . Our extension of this technique sets the ground for a number of exciting studies beyond a chip-based approach. In particular, the ease of tuning the trap stiffness in real time allows on-command capture, displacement and release of nanoparticles by simply moving the nanopipette. Furthermore, the open architecture of the approach allows manipulation of charged nanoparticles away from macroscopic substrates provided that a counter surface larger than a few hundred nanometres is available, for example, a micron-sized bead [28] . Moreover, the nanopipette may be used for in situ local introduction of chemicals to control ion strength, pH, or other ingredients that are crucial for the trapped particle. These features make this trapping geometry generally suitable for studying the interaction of a nanoparticle with other molecules in confined spaces and at surfaces, where short-range phenomena such as catalytic or plasmonic effects are at work. In our current article, we demonstrate applications in lipid membrane biophysics with future prospects in probing membrane heterogeneity [29] , [30] and nanoscopic interactions with vesicles, viruses and protein complexes. Another exciting and challenging future direction will be the realization of traps in physiological buffer. A scannable aperture or indentation (for example, at the end of an AFM tip) could facilitate this goal because trap parameters can be adjusted more easily than for nanofabricated substrates. Indeed, the trap stiffness of k r =0.097 pN nm −1 presented in this work is already higher than te previous reports of electrostatic fluidic traps [8] . Sample preparation Glass nanopipettes with 114±54 nm inner diameter and 562±68 nm outer diameter were fabricated by a multi-step pulling process using a laser-based pipette puller (P-2000, Sutter Instrument). The nanopipettes were cleaned by standard rinsing and an O 2 plasma process. The pipette was dipped into deionized water about 20 min to minimize its capillary rise effect. Samples of 60-nm and 40-nm gold nanospheres (British Biocell International) were centrifuged and resuspended in deionized water (18 MΩ cm −1 ) twice to remove traces of salt or other contaminants. Small unilamellar vesicles were prepared by extrusion. Briefly, the lipid mixture containing 86.6 mol% DOPC, Avanti Polar Lipids, 13 mol% 1,2-dioleoyl-sn-glycero-3-phospho-(1′-rac-glycerol) (DOPG, Avanti Polar Lipids) and 0.4 mol% Atto532-DOPE (ATTO-TEC GmbH) was dried under clean dry nitrogen and rehydrated in deionized water, vortexed and extruded through 50 nm polycarbonate membranes (Avestin). The charge values of the sample particles were obtained from zeta-potential measurements by means of light scattering. Supported lipid membranes consisting of DOPC doped with 1 mol% ganglioside GM1 (Avanti Polar Lipids) and trace amounts ( ⩽ 0.1 mol%) of Atto532-DOPE were prepared by vesicle fusion and spreading on a glass substrate [27] . The final ion strengths in the aqueous solutions were ~4 × 10 −5 M. For the experiments on anchored vesicles, supported membranes consisting of DOPC and 0.2 mol% Biotinyl Cap PE were prepared. After incubation with avidin solution for 5 min, unbound avidin was removed by washing. Biotinylated small unilamellar vesicles consisting of 94.4 mol% DOPC, 5 mol% trisialoganglioside (GT1b, Sigma-Aldrich), 0.2 mol% Biotinyl Cap PE, and 0.4 mol% Atto532-DOPE (ATTO-TEC GmbH) were added to the supported lipid membrane in deionized water environment. Scattering interferometry GNPs (60 nm, 40 nm) were imaged by iSCAT with a high three-dimensional localization accuracy of ⩽ 5 nm at 1.9 kHz. A 30 mW diode-pumped solid-state laser (TECGL-30, WSTech) at λ =532 nm, near the plasmon resonance wavelength of a typical GNP, was focused onto the sample by a × 100, 1.3 NA oil immersion objective (Zeiss). The scattered and reflected lights were collected by the objective and imaged on a CMOS camera (MV-D1024-160-CL-12, PhotonFocus) at an acquisition rate of 1.9 kHz. The peak position and the height of the iSCAT image point-spread function yield the transverse ( x – y ) and vertical ( z ) positions of the confined particle, respectively. To calibrate the iSCAT contrast as a function of the particle's vertical position [19] , we attached a particle to the end of a nanopipette and recorded its contrast at different heights. The detailed procedure of handling iSCAT images, for example, correcting for the background caused by the nanopipette, can be found in ref. 19 . Scanning a nanopipette The position of a nanopipette in a liquid chamber was controlled with a 3-axis piezo scanner (TRITOR 38, Piezosystem Jena). The scanning system had a high spatial stability of ⩽ 2 nm during a typical measurement time of ~1 s. The pipette-substrate gaps was precisely controlled with iSCAT detection. We detected the contact point between the pipette and the substrate by monitoring the interference of the light scattered by the nanopipette and reflected by the substrate during step-wise approaching (~10 nm). When the pipette touched the substrate, the interferometric signal did not change further in one step approaching of the pipette. To get a specific pipette-substrate gaps in the range of 100~300 nm, the pipette was pulled back again by the piezo scanner. We note that in our current work, the tip-sample distance was not actively stabilized. However, this can be done with nanometre accuracy by using shear-force distance regulation, which is common in scanning near-field microscopy (see for example, ref. 31 ). Fluorescence imaging Fluorescence-labelled lipid vesicles with diameter 50 nm were imaged in a standard wide-field configuration using 532 nm excitation and a 545 long-pass filter. Images were obtained at an acquisition rate of 25 frames per second using a × 100, 1.3 NA oil immersion objective (Zeiss) and a CCD camera (Watec 120N). How to cite this article : Kim, J. T. et al. Scanning-aperture trapping and manipulation of single charged nanoparticles. Nat. Commun. 5:3380 doi: 10.1038/ncomms4380 (2014).